TRIM29 regulates the assembly of DNA repair proteins into damaged chromatin Although DNA double-strand break (DSB) repair is mediated by numerous proteins accumulated at DSB sites, how DNA repair proteins are assembled into damaged chromatin has not been fully elucidated. Here we show that a member of the tripartite motif protein family, TRIM29, is a histone-binding protein responsible for DNA damage response (DDR). We found that TRIM29 interacts with BRCA1-associated surveillance complex, cohesion, DNA-PKcs and components of TIP60 complex. The dynamics of the TRIM29-containing complex on H2AX nucleosomes is coordinated by a cross-talk between histone modifications. TRIM29 binds to modified histone H3 and H4 tails in the context of nucleosomes. Furthermore, chromatin binding of TRIM29 is required for the phosphorylation of H2AX and cell viability in response to ionizing radiation. Our results suggest that TRIM29 functions as a scaffold protein to assemble DNA repair proteins into chromatin followed by efficient activation of DDR. DNA double-strand break (DSB) is a serious DNA lesion that is caused by various genotoxic stresses including ionizing radiation (IR), DNA replication errors and alkylating reagents. Deficiency or inaccuracy of DSB repair leads to various diseases including cancer, neurodegeneration and immunodeficiency [1] . To overcome the intense toxicity of DSBs and maintain genome stability, cells have developed elaborate surveillance mechanisms to detect DNA lesions and recruit DNA repair proteins to the DSB sites [2] . In the first step of DDR, the MRE11-RAD50-NBS1 (MRN) complex and Ku70-Ku80 heterodimer bind to the DSB ends and activate ATM and DNA-PKcs, respectively [3] , [4] . Then histone H2AX at Ser 139 is rapidly phosphorylated by ATM and DNA-PKcs in response to DSBs [5] . Following the induction of phosphorylated H2AX at Ser 139 (γH2AX), many regulators of the DNA repair pathway accumulate at DSB sites and activate the DSB repair pathway [6] , [7] . In addition to these sensor factors of DSBs, various proteins contribute to the DSB repair pathway. MSH2 and MSH6 have a fundamental role in promoting DNA mismatch repair (MMR) and are also involved in the recruitment of DSB repair factors to the DSB sites [8] . Several DNA repair factors form a multiprotein complex. For example, ATM, MRN complex and MSH2-MSH6 dimer are components of the BRCA1-associated surveillance complex (BASC) [9] . Cooperative assembly of DNA repair proteins into chromatin plays a critical role in the maintenance of chromatin integrity. Accumulating evidence indicates that a variety of histone modifications function as a molecular switch in the recruitment of DSB repair proteins to the DSB sites [10] , [11] . Dimethylated H4 at Lys 20 (H4K20me2) facilitates the accumulation of 53BP1 at the DSB sites [12] , [13] . Conversely, acetylation of H4 at Lys 16 (H4K16Ac) by TIP60 promotes the accumulation of BRCA1 by inhibiting the recruitment of 53BP1 to the DSB sites [13] . Dimethylated H3 at Lys 36 (H3K36me2) recruits NBS1 and Ku70 at the DSB sites [14] . SETD2-dependent trimethylated H3K36 (H3K36me3) plays an important role in both DSB repair and the MMR pathway [15] , [16] , [17] . The assembly of DNA repair proteins into chromatin is coordinated by a cross-talk between posttranslational modifications (PTMs) of histones. The gene encoding ATM is responsible for ataxia telangiectasia (AT), which is an autosomal recessive disorder with pleiotropic phenotypes, including neuronal degeneration, immune dysfunction, premature ageing and increased cancer risk [18] . Tripartite motif protein 29 ( TRIM29 ) was identified as an AT group D-complementing gene in a functional complementation study with an AT cell line by transfection with a human cosmid library [19] . The TRIM protein family is characterized by the presence of a tripartite motif composed of a RING finger domain, one or two B-box domains and a coiled-coil domain [20] . Knockdown of TRIM29 in SiHa, Panc1 and BxPC3 cell lines increased radiosensitivity [21] , [22] . Moreover, phosphorylation of TRIM29 by ATM and MAPKAP kinase 2 (MK2) contributes to the radioresistance of cells [22] . Although TRIM29 has been shown to interact with several proteins including protein kinase C substrate, disheveled-2, p53 and TIP60 (refs 21 , 23 , 24 , 25 ), little is known about how TRIM29 enhances the radioresistance of cells. Here we show that TRIM29 is a histone-binding protein involved in the regulation of DDR. Our biochemical studies reveal that TRIM29 forms a multiprotein complex with BASC components, cohesion, DNA-PKcs and TIP60 complex. The dynamics of the TRIM29 complex on nucleosomes containing H2AX are coordinated by H3K36me2/3, H4K16Ac and H4K20me2. Chromatin binding of TRIM29 is also required to promote DDR. We propose that TRIM29 functions as a scaffold protein incorporating DNA repair proteins into chromatin and contributes to efficient activation of DNA damage signalling. TRIM29 forms a protein complex with DNA repair proteins To clarify which types of cells express TRIM29, we performed western blot analysis with the lysates of several cell lines. Consistent with the prediction using RefExA and previous reports [26] , TRIM29 was highly expressed in epithelial cancer cell lines including HeLa, HeLa S3 and SiHa cells but not in HEK293T and U2OS cells ( Supplementary Fig. 1a ). Although exogenous TRIM29 has been shown to be localized in the cytoplasm [27] , the subcellular localization of endogenous TRIM29 remains to be elucidated. We fractionated the lysates of HeLa S3, HeLa and SiHa cells into cytoplasmic, nucleoplasmic and chromatin fractions as shown in Fig. 1a [28] and determined the subcellular localization of TRIM29. Both full-length TRIM29 and a truncated variant of TRIM29 with a molecular weight of about 50 kDa were expressed in the chromatin fraction ( Fig. 1b and Supplementary Fig. 1b ). The truncated variant is likely to be an amino-terminal truncated variant and to be translated from the internal start codon methionine 143. Indeed, an N-terminal truncated variant that shares 99% homology with full-length TRIM29 residues Met 143 to Pro 588 has already been isolated [29] . Immunofluorescence staining of endogenous TRIM29 revealed that the distribution of TRIM29 overlapped with the 4,6-diamidino-2-phenylindole (DAPI)-stained region of chromatin in HeLa S3 cells ( Fig. 1c ). TRIM29 knockdown in HeLa S3, HeLa and SiHa cells decreased immunofluorescence signals of TRIM29 in the DAPI-stained region ( Supplementary Fig. 1c,d ). Next, we generated HeLa S3 and U2OS cells stably expressing carboxy-terminal enhanced green fluorescent protein (EGFP)-tagged TRIM29 and investigated whether it is located on chromatin. The distribution of TRIM29-EGFP was overlapped with the DAPI-stained region in HeLa S3 cells but not in U2OS cells ( Supplementary Fig. 1e ). These findings indicate that TRIM29 is located on chromatin in epithelial cancer cells. 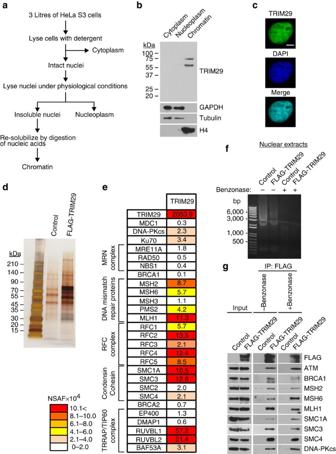Figure 1: TRIM29 binds to DNA DSB repair proteins. (a) Outline of the preparation of cytoplasm, nucleoplasm and chromatin fractions. (b) Subcellular localization of endogenous TRIM29 in HeLa S3 cells. Total proteins (10 μg) from the cytoplasm, nucleoplasm and chromatin fractions were subjected to SDS–PAGE followed by western blotting. (c) Confocal immunofluorescence images showing the localization of endogenous TRIM29 in HeLa S3 cells. DNA was counterstained with DAPI. Scale bar, 5 μm. (d) Silver staining of the TRIM29-containing protein complex immunopurified from HeLa S3 cells stably expressing FLAG-tagged TRIM29 on 4%–20% gradient SDS–PAGE gel. (e) List of TRIM29-associated proteins identified by MudPIT. See alsoSupplementary Table 1. (f) Agarose gel electrophoresis (1% w/v) showing nucleic acids of benzonase-treated or -untreated nuclear extracts prepared from FLAG-TRIM29-expressing HeLa S3 cells. (g) Western blot analysis of immunopurified proteins with FLAG-tagged TRIM29 from nuclear extracts after treatment without or with benzonase. Figure 1: TRIM29 binds to DNA DSB repair proteins. ( a ) Outline of the preparation of cytoplasm, nucleoplasm and chromatin fractions. ( b ) Subcellular localization of endogenous TRIM29 in HeLa S3 cells. Total proteins (10 μg) from the cytoplasm, nucleoplasm and chromatin fractions were subjected to SDS–PAGE followed by western blotting. ( c ) Confocal immunofluorescence images showing the localization of endogenous TRIM29 in HeLa S3 cells. DNA was counterstained with DAPI. Scale bar, 5 μm. ( d ) Silver staining of the TRIM29-containing protein complex immunopurified from HeLa S3 cells stably expressing FLAG-tagged TRIM29 on 4%–20% gradient SDS–PAGE gel. ( e ) List of TRIM29-associated proteins identified by MudPIT. See also Supplementary Table 1 . ( f ) Agarose gel electrophoresis (1% w/v) showing nucleic acids of benzonase-treated or -untreated nuclear extracts prepared from FLAG-TRIM29-expressing HeLa S3 cells. ( g ) Western blot analysis of immunopurified proteins with FLAG-tagged TRIM29 from nuclear extracts after treatment without or with benzonase. Full size image To understand the function of TRIM29 in chromatin, we generated HeLa S3 cells stably expressing FLAG-TRIM29, prepared nuclear extracts from the cells by Dignam’s method and then immunopurified FLAG-TRIM29 and TRIM29-associated proteins from the nuclear extracts ( Fig. 1d ). We identified many of TRIM29-binding proteins by multidimensional protein identification technology (MudPIT) mass spectrometry. The relative abundance of a particular protein was assessed by means of a normalized spectral abundance factor, or NSAF [30] . MudPIT analysis revealed that TRIM29 formed a multiprotein complex with DSB repair proteins ( Fig. 1e and Supplementary Table 1 ). Many of these proteins have DNA-binding activity, raising the possibility that formation of the TRIM29 complex is dependent on DNA derived from nuclear extracts. To exclude this possibility, we treated nuclear extracts with benzonase, immunopurified TRIM29-binding proteins and then analysed TRIM29-associated proteins. Agarose gel electrophoresis of the nuclear extracts revealed that nuclear extracts did not contain DNA ( Fig. 1f ). Western blotting and silver staining showed that the TRIM29 complex can be formed independently of DNA ( Fig. 1g and Supplementary Fig. 2a ). We also found that TRIM29 was copurified with ATM ( Fig. 1g ). BASC, DNA-PKcs, cohesin and TIP60 complex play an important role in DDR [5] , [10] , [31] , [32] , suggesting that formation of the TRIM29 complex is dependent on genotoxic stress. To address this possibility, we purified the TRIM29 complex from nuclear extracts of cells treated with or without IR and analysed TRIM29-associated proteins. There was no significant difference in composition of the TRIM29 complex after IR treatment ( Supplementary Fig. 2b,c ). Interaction of TRIM29 with DNA repair proteins To identify the region of TRIM29 necessary for interaction with DNA repair and other proteins, we generated HeLa S3 cells stably expressing the series of truncated mutants of FLAG-TRIM29 diagrammed in Fig. 2a . Western blotting and MudPIT analysis showed that TRIM29-associated proteins were copurified with the truncated mutant of 394-588 but not with truncate 470-588 ( Fig. 2b , Supplementary Fig. 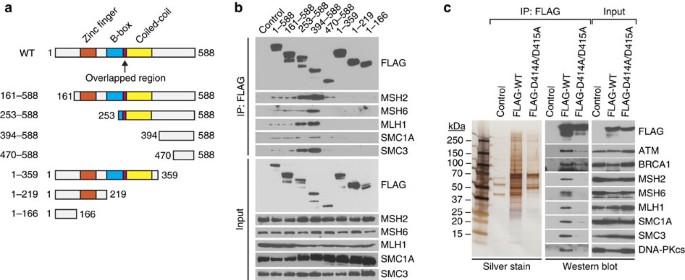Figure 2: C-terminal region of TRIM29 is required for binding to DNA repair proteins. (a) Schematic representation of WT TRIM29 and truncated mutant proteins. (b) Western blot analysis of proteins associated with WT TRIM29 and mutants. Anti-FLAG immunoprecipitates were prepared from nuclear extracts after treatment with benzonase and analysed by western blotting. (c) Western blot analysis of proteins associated with FLAG-tagged WT TRIM29 and D414A/D415A mutant in which D414 and D415 were substituted with alanine. 2d and Supplementary Table 2 ). 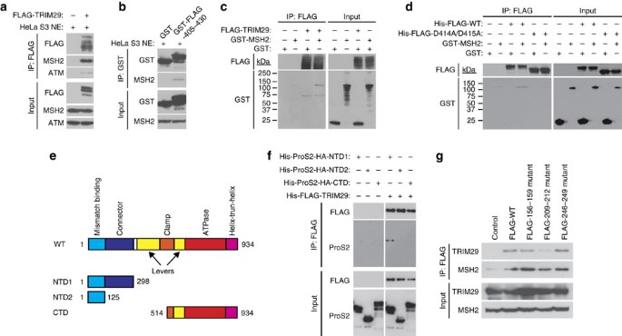Figure 3: TRIM29 directly binds to MSH2. (a) Western blot analysis of proteins pulled down by recombinant FLAG-tagged TRIM29 from nuclear extracts of HeLa S3 cells. FLAG-tagged TRIM29 attached to M2-agarose was incubated with nuclear extracts from HeLa S3 cells. The bound proteins were washed and eluted by 3 × FLAG peptides and analysed by western blotting. (b) Western blot analysis of proteins pulled down by recombinant GST-FLAG-tagged TRIM29 peptide (residues 405–430) from nuclear extracts of HeLa S3 cells. GST-FLAG-405-430 attached to GST-Sepharose was incubated with nuclear extracts from HeLa S3 cells and washed. The binding proteins were eluted by glutathione and analysed by western blotting. (c) Direct binding of His-FLAG-TRIM29 to GST-MSH2. His-FLAG-TRIM29 attached to M2-agarose was incubated with GST or GST-MSH2. The bound proteins were washed and eluted by 3 × FLAG peptides followed by western blotting. (d)In-vitropull-down assay of GST-MSH2 with WT His-FLAG-TRIM29 or D414A/D415A mutant in which D414 and D415 were substituted with alanine. Anti-FLAG pull-down assay was performed as described ina. (e) Schematic representation of WT MSH2 and mutant proteins. (f) Direct binding of WT His-FLAG-TRIM29 and mutants to His-ProS2-HA-MSH2. Anti-FLAG pull-down assay was performed as described ina. (g) Western blot analysis of FLAG-tagged immunoprecipitates from HeLa S3 cells stably expressing WT FLAG-tagged MSH2 and mutants in which residues 156–159, 209–212 and 246–249 were substituted with alanine. Secondary structure prediction by PSIPRED ( http://bioinf.cs.ucl.ac.uk/psipred/ ) revealed that the region of amino acid residues from 405 to 430 was highly conserved among the species ( Supplementary Table 3 ). To determine whether the region is critical for formation of the TRIM29 complex, we generated HeLa S3 cells stably expressing FLAG-TRIM29 D414A/D415A in which Asp414 and Asp415 are substituted with Ala. Although D414A/D415A mutations interfered with TRIM29 binding to components such as MSH2/MSH6 in the complex, ATM and BRCA1 still interacted with the D414A/D415A mutant ( Fig. 2c ). Thus, the C-terminal region is required for interaction of TRIM29 with some DNA repair proteins including MSH2/MSH6 but not for interaction with ATM and BRCA1. Figure 2: C-terminal region of TRIM29 is required for binding to DNA repair proteins. ( a ) Schematic representation of WT TRIM29 and truncated mutant proteins. ( b ) Western blot analysis of proteins associated with WT TRIM29 and mutants. Anti-FLAG immunoprecipitates were prepared from nuclear extracts after treatment with benzonase and analysed by western blotting. ( c ) Western blot analysis of proteins associated with FLAG-tagged WT TRIM29 and D414A/D415A mutant in which D414 and D415 were substituted with alanine. Full size image TRIM29 directly binds to MSH2 To determine which protein in the complex directly binds to TRIM29, we performed an in-vitro binding assay using recombinant FLAG-TRIM29 protein and HeLa S3 nuclear extracts. We found that FLAG-TRIM29 copurified with MSH2 and ATM ( Fig. 3a ). We next performed an in-vitro binding assay of the GST-TRIM29 peptide (residues 405–430) with HeLa S3 nuclear extracts. GST-TRIM29 peptide interacted with MSH2, but not with glutathione S -transferase (GST) alone ( Fig. 3b ). As expected, GST-MSH2 interacted with full-length TRIM29, but GST alone did not ( Fig. 3c ). D414A/D415A mutations in TRIM29 interfered with direct interaction of TRIM29 with MSH2 ( Fig. 3d ). We examined which region in MSH2 is responsible for direct interaction with TRIM29. We produced recombinant MSH2 mutants shown in Fig. 3e and performed an in-vitro binding assay with FLAG-TRIM29 and a series of truncated mutants of MSH2. As shown in Fig. 3f , only NTD1 bound to TRIM29, indicating that the connector domain of MSH2 directly binds to TRIM29. Previously, it was shown that the connector domain of MSH2 has three surface loops consisting of amino acids residues 150–160, 207–217 and 243–262 that are not conserved in prokaryotic MutS [33] . To test the possibility that TRIM29 interacts with MSH2 through these loops, we generated HeLa S3 cells stably expressing three kinds of FLAG-MSH2 mutants in which amino acids residues 156–159, 209–212 and 246–249 were substituted with alanine, respectively. Point mutations of residues 209–212 disrupted the interaction with TRIM29 ( Fig. 3g ), suggesting that TRIM29 directly binds to the surface loop from 207 to 217 of MSH2. Figure 3: TRIM29 directly binds to MSH2. ( a ) Western blot analysis of proteins pulled down by recombinant FLAG-tagged TRIM29 from nuclear extracts of HeLa S3 cells. FLAG-tagged TRIM29 attached to M2-agarose was incubated with nuclear extracts from HeLa S3 cells. The bound proteins were washed and eluted by 3 × FLAG peptides and analysed by western blotting. ( b ) Western blot analysis of proteins pulled down by recombinant GST-FLAG-tagged TRIM29 peptide (residues 405–430) from nuclear extracts of HeLa S3 cells. GST-FLAG-405-430 attached to GST-Sepharose was incubated with nuclear extracts from HeLa S3 cells and washed. The binding proteins were eluted by glutathione and analysed by western blotting. ( c ) Direct binding of His-FLAG-TRIM29 to GST-MSH2. His-FLAG-TRIM29 attached to M2-agarose was incubated with GST or GST-MSH2. The bound proteins were washed and eluted by 3 × FLAG peptides followed by western blotting. ( d ) In-vitro pull-down assay of GST-MSH2 with WT His-FLAG-TRIM29 or D414A/D415A mutant in which D414 and D415 were substituted with alanine. Anti-FLAG pull-down assay was performed as described in a . ( e ) Schematic representation of WT MSH2 and mutant proteins. ( f ) Direct binding of WT His-FLAG-TRIM29 and mutants to His-ProS2-HA-MSH2. Anti-FLAG pull-down assay was performed as described in a . ( g ) Western blot analysis of FLAG-tagged immunoprecipitates from HeLa S3 cells stably expressing WT FLAG-tagged MSH2 and mutants in which residues 156–159, 209–212 and 246–249 were substituted with alanine. Full size image TRIM29 interacts with components of the TIP60 complex We previously identified TIP60 as one of the TRIM29-interacting proteins [24] . MudPIT analysis also revealed that FLAG-TRIM29 is copurified with some components of the TIP60 complex including EP400, DMAP1, RUVBL1 and BAF53 ( Fig. 1e ). Thus, we investigated whether TRIM29 is copurified with some components of the TIP60 complex. RUVBL1 and BAF53a, but not BAF53b, were copurified with TRIM29 ( Supplementary Fig. 3a ). To address reciprocal interactions of the TIP60 complex with TRIM29, we generated HeLa S3 cells stably expressing FLAG-TIP60, DMAP1 and ING3, which are components of the TIP60 complex. TIP60, DMAP1 and ING3 were copurified with TRIM29 ( Supplementary Fig. 3b,c,d ). To test whether TRIM29 directly binds to the TIP60 complex, we performed an in-vitro binding assay using recombinant TRIM29 and the TIP60 complex purified from cells expressing FLAG-TIP60. TRIM29 did not directly bind to the TIP60 complex ( Supplementary Fig. 3e ). These findings suggest that TRIM29 indirectly interacts with the TIP60 complex. TRIM29 is required for activation of DDR The constitutive interaction of TRIM29 with ATM, DNA-PKcs and TIP60 suggests that TRIM29 is also one of the regulators in the DSB repair pathway. To examine whether TRIM29 regulates histone PTMs in response to DSBs, we knocked down TRIM29 in HeLa S3 cells by small interfering RNA (siRNA) transfection, treated the cells with 10 Gy and then analysed IR-induced histone PTMs. TRIM29 depletion decreased the basal level of γH2AX ( Fig. 4a,b and Supplementary Fig. 4a ), indicating that TRIM29 regulates the basal level of γH2AX. TRIM29-depleted cells showed a lower level of IR-induced γH2AX than did siCTRL-treated cells ( Fig. 4a,b ). TRIM29 knockdown did not show any significant difference in the level of other histone modifications in response to IR treatment ( Fig. 4a,c ). We examined the level of γH2AX at the indicated time points from 0 to 120 min and 0 to 24 h after IR treatment. TRIM29 depletion caused a decrease in the level of global γH2AX at the indicated time points ( Fig. 4d and Supplementary Fig. 4b ). Consistent with the defect of γH2AX and H4K16Ac signals in TRIM29-depleted cells, TRIM29 knockdown caused a reduction in radioresistance ( Fig. 4e ). 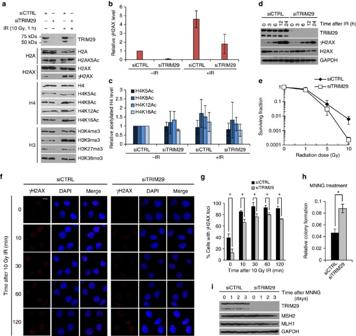Figure 4: TRIM29 regulates DNA DDR. (a) Effect of TRIM29 knockdown on histone modifications induced by IR treatment. TRIM29-depleted HeLa S3 cells were treated with 10 Gy IR and collected after 1 h. Histones were analysed by western blotting. (b,c) Intensities of γH2AX and acetylated H4 normalized with the values of H2AX and H4, respectively. Band intensities were quantified using NIH ImageJ software. Three independent experiments were performed. Error bars show s.d. (d) Effects of TRIM29 knockdown on the phosphorylation of H2AX. TRIM29-depleted HeLa S3 cells were treated with 10 Gy IR and collected at the indicated time points from 0 to 24 h after IR treatment. Whole-cell lysates were analysed by western blotting. (e) Survival curves of TRIM29-depleted HeLa S3 cells. Three independent experiments were performed. (f) Effect of TRIM29 knockdown on the formation of γH2AX foci. TRIM29-depleted HeLa S3 cells were treated with 10 Gy, fixed at the indicated time points from 0 to 120 min after IR treatment and stained with anti-γH2AX antibody. DNA was counterstained with DAPI. Scale bar, 10 μm. (g) Percentages of γH2AX foci-positive cells (> 10 foci per nucleus) from the data shown inf. Three independent experiments in which at least 30 cells were counted were performed.P-values were determined by Student’st-test (*P<0.05). Error bars show s.d. (h) Effect of MNNG on viability of TRIM29-depleted cells. TRIM29-depleted HeLa S3 cells were treated with 10 μM MNNG for 2 h. Cell viability in response to MNNG treatment was analysed by a colony-formation assay.P-values were determined by Student’st-test (*P<0.05). Three independent experiments were performed. Error bars show s.d. (i) Effect of TRIM29 knockdown on the stability of MSH2 and MLH1 under the condition of MNNG treatment. TRIM29-depleted HeLa S3 cells were treated with 10 μM MNNG for 2 h and collected at 0, 1, 2 and 3 days. Whole-cell lysates were analysed by western blotting. Figure 4: TRIM29 regulates DNA DDR. ( a ) Effect of TRIM29 knockdown on histone modifications induced by IR treatment. TRIM29-depleted HeLa S3 cells were treated with 10 Gy IR and collected after 1 h. Histones were analysed by western blotting. ( b , c ) Intensities of γH2AX and acetylated H4 normalized with the values of H2AX and H4, respectively. Band intensities were quantified using NIH ImageJ software. Three independent experiments were performed. Error bars show s.d. ( d ) Effects of TRIM29 knockdown on the phosphorylation of H2AX. TRIM29-depleted HeLa S3 cells were treated with 10 Gy IR and collected at the indicated time points from 0 to 24 h after IR treatment. Whole-cell lysates were analysed by western blotting. ( e ) Survival curves of TRIM29-depleted HeLa S3 cells. Three independent experiments were performed. ( f ) Effect of TRIM29 knockdown on the formation of γH2AX foci. TRIM29-depleted HeLa S3 cells were treated with 10 Gy, fixed at the indicated time points from 0 to 120 min after IR treatment and stained with anti-γH2AX antibody. DNA was counterstained with DAPI. Scale bar, 10 μm. ( g ) Percentages of γH2AX foci-positive cells (> 10 foci per nucleus) from the data shown in f . Three independent experiments in which at least 30 cells were counted were performed. P -values were determined by Student’s t -test (* P <0.05). Error bars show s.d. ( h ) Effect of MNNG on viability of TRIM29-depleted cells. TRIM29-depleted HeLa S3 cells were treated with 10 μM MNNG for 2 h. Cell viability in response to MNNG treatment was analysed by a colony-formation assay. P -values were determined by Student’s t -test (* P <0.05). Three independent experiments were performed. Error bars show s.d. ( i ) Effect of TRIM29 knockdown on the stability of MSH2 and MLH1 under the condition of MNNG treatment. TRIM29-depleted HeLa S3 cells were treated with 10 μM MNNG for 2 h and collected at 0, 1, 2 and 3 days. Whole-cell lysates were analysed by western blotting. Full size image To confirm that TRIM29 regulates the formation of γH2AX foci, we knocked down TRIM29 in HeLa S3 cells by siRNA transfection, treated the cells with 10 Gy and analysed the formation of γH2AX foci at the indicated time points from 0 to 120 min after IR treatment. TRIM29 depletion reduced the number of γH2AX foci at all of the indicated times ( Fig. 4f,g ). We speculated that the formation of γH2AX foci induced even without IR treatment is due to spontaneous DNA damage or chromosome instability. To determine the role of TRIM29 in the formation of γH2AX foci, we analysed the localization of TRIM29 in response to IR-induced DSBs. TRIM29 did not accumulate at γH2AX foci ( Supplementary Fig. 4c ). We obtained similar results using ectopically N-terminal or C-terminal EGFP-tagged TRIM29-expressing HeLa S3 cells ( Supplementary Fig. 4d ). These findings suggest that TRIM29 regulates the induction of γH2AX in response to DNA damage. We found that TRIM29 directly binds to MSH2, which is a key regulator of the MMR pathway [8] , raising the possibility that TRIM29 regulates the MMR pathway ( Fig. 3 ). It has been reported that MSH2- and MLH1-deficient cells are highly resistant to N -methyl- N ′-nitro- N -nitrosoguanidine (MNNG) and show increased viability in response to MNNG [34] . We therefore analysed the effect of MNNG treatment on the viability of TRIM29-depleted HeLa S3 cells. TRIM29 depletion increased the viability of cells subjected to MNNG treatment ( Fig. 4h ). To determine whether the resistance of TRIM29-depleted cells to MNNG is due to the defect of MSH2 and MLH1, we analysed the effect of TRIM29 depletion and the effect of MNNG treatment on protein expression of MSH2 and MLH1. Both MSH2 and MLH1 were stably expressed in TRIM29 siRNA- and/or MNNG-treated HeLa S3 cells ( Fig. 4i ). These observations demonstrate that MNNG resistance of the cells is due to the absence of TRIM29. Taken together, these results suggest that TRIM29 functions upstream of both the DSB repair and MMR pathways. Histone PTMs regulate interaction of TRIM29 with H2AX To investigate how the TRIM29 complex interacts with H2AX nucleosomes, we generated HeLa S3 cells stably expressing FLAG-H2AX wild type (WT) or S139A mutant in which Ser139 was substituted with alanine, and we purified histones containing FLAG-H2AX WT or S139A mutant from nuclear extracts of cells treated with or without 10 Gy IR. For this analysis, we treated nuclear extracts with nuclease to exclude DNA–protein interactions. Silver staining showed that both WT and S139A of H2AX copurified all four core histones ( Fig. 5a ). TRIM29 and other components of the TRIM29 complex bound to histones containing H2AX ( Fig. 5b ). Although FLAG-H2AX was phosphorylated even without IR treatment, this may be due to spontaneous DNA damage and genome instability. IR treatment caused a moderate decrease in the interactions of TRIM29, MSH6 and MLH1 with γH2AX ( Fig. 5b ). Consistent with the previous findings that ATM, BRCA1, SMC1A and SMC3 are accumulated at DSB sites in a γH2AX-dependent manner, IR treatment caused an increase in the interactions of ATM, BRCA1, SMC1A and SMC3 with γH2AX ( Fig. 5b ). S139A mutation of H2AX reduced the interaction of TRIM29 with histones containing H2AX but did not completely abrogate the interaction, suggesting that other histone modifications also contribute to the binding of TRIM29 to H2AX-containing nucleosomes ( Fig. 5b ). S139A mutation of H2AX abrogated interaction of BASC subunits and DNA-PKcs with histones, whereas SMC1A and SMC3 interacted with histones regardless of S139A mutation ( Fig. 5b ). Taken together, these findings suggest that dissociation of TRIM29 and MMR proteins from γH2AX-containing histones promotes the accumulation of ATM, BRCA1 and cohesin in γH2AX foci. 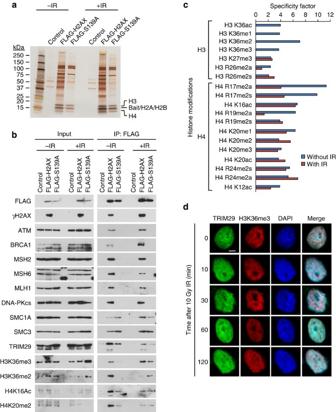Figure 5: TRIM29 is located on nucleosomes containing H2AX. (a) Silver staining of anti-FLAG immunoprecipitates from nuclear extracts of cells expressing FLAG-tagged WT H2AX and S139 mutant on 4%–20% gradient SDS–PAGE gel. (b) Western blot analysis of proteins associated with FLAG-tagged WT H2AX and S139A mutant. HeLa S3 cells expressing FLAG-tagged WT H2AX and S139A mutant were untreated or treated with 10 Gy IR. After 1 h, FLAG-tagged immunoprecipitates were prepared from each cell line. (c) Binding specificity of FLAG-tagged TRIM29 to modified histone peptides using Modified Histone Peptide Arrays. FLAG-tagged TRIM29 complex was prepared from HeLa S3 cells expressing FLAG-TRIM29 untreated or treated with 10 Gy IR for 1 h. This experiment was performed according to the manufacturer’s protocol. (d) Immunofluorescence images showing the localization of TRIM29 and H3K36me3. HeLa S3 cells were treated with 10 Gy IR, fixed at the indicated time points from 0 to 120 min and stained with anti-TRIM29 and H3K36me3 antibodies. DNA was counterstained with DAPI. Scale bar, 5 μm. Figure 5: TRIM29 is located on nucleosomes containing H2AX. ( a ) Silver staining of anti-FLAG immunoprecipitates from nuclear extracts of cells expressing FLAG-tagged WT H2AX and S139 mutant on 4%–20% gradient SDS–PAGE gel. ( b ) Western blot analysis of proteins associated with FLAG-tagged WT H2AX and S139A mutant. HeLa S3 cells expressing FLAG-tagged WT H2AX and S139A mutant were untreated or treated with 10 Gy IR. After 1 h, FLAG-tagged immunoprecipitates were prepared from each cell line. ( c ) Binding specificity of FLAG-tagged TRIM29 to modified histone peptides using Modified Histone Peptide Arrays. FLAG-tagged TRIM29 complex was prepared from HeLa S3 cells expressing FLAG-TRIM29 untreated or treated with 10 Gy IR for 1 h. This experiment was performed according to the manufacturer’s protocol. ( d ) Immunofluorescence images showing the localization of TRIM29 and H3K36me3. HeLa S3 cells were treated with 10 Gy IR, fixed at the indicated time points from 0 to 120 min and stained with anti-TRIM29 and H3K36me3 antibodies. DNA was counterstained with DAPI. Scale bar, 5 μm. Full size image H3K36me2/3, H4K16Ac and H4K20me2 function as molecular scaffolds for DNA repair proteins [13] , [15] , [17] . We therefore investigated whether the dynamics of the TRIM29 complex on H2AX nucleosomes is correlated with H3K36me2/3, H4K16Ac and H4K20me2. IR-induced phosphorylation of H2AX led to a decrease in the amounts of TRIM29, H3K36me2, H4K16Ac and H4K20me2 in the H2AX-containing nucleosomes and an increase in the amount of H3K36me3 ( Fig. 5b ). These findings suggest that interaction of the TRIM29 complex with H2AX nucleosomes is regulated by histone PTMs. To determine which histone modifications contribute to the interaction of the TRIM29 complex with histones, we performed an in-vitro binding assay using modified histone tail peptide arrays containing various combinations of modifications on the N-terminal tails of core histones. Consistent with the results showing that the amount of the TRIM29 complex on H2AX nucleosomes is correlated with that of H3K36me2/3, H4K16Ac and H4K20me2 ( Fig. 5b ), the TRIM29 complex showed high affinity to modified H4 tails (residues 16 to 20) and H3K36 ( Fig. 5c ). Although the TRIM29 complex purified from IR-treated cells expressing FLAG-TRIM29 exhibited high affinity to modified H4 tails (residues 16 to 20), binding level of the TRIM29 complex to modified H4 tails was not greatly affected by DNA damage. In contrast, we observed remarkable reduction of TRIM29 complex binding to modified H3K36 after DNA damage in vitro ( Fig. 5c ). Consistent with the results showing that the TRIM29 complex binds to H3 tails with H3K36me, TRIM29 was partially colocalized with H3K36me3; however, IR treatment did not affect the localization of TRIM29 with H3K36 ( Fig. 5d ). Therefore, other modifications of histones may also contribute to regulation of the level of TRIM29 interacting with the nucleosomes in cells. These findings suggest that assembly of the TRIM29 complex on γH2AX-containing nucleosomes is regulated by a cross-talk between modified H3 and H4. TRIM29 interacts with modified histone tails To identify the binding domain of TRIM29 to chromatin, we prepared nucleosome-enriched extracts from cells expressing full-length (1–588) and truncated mutants (161–588, 253–588 and 1–219) of FLAG-TRIM29 using MNase, because nuclear extracts prepared by Dignam’s method contain few nucleosomes. Full-length TRIM29 copurified with H3, whereas each mutant did not, suggesting that both N-terminal and C-terminal regions of TRIM29 are required for binding to nucleosomes ( Fig. 6a ). 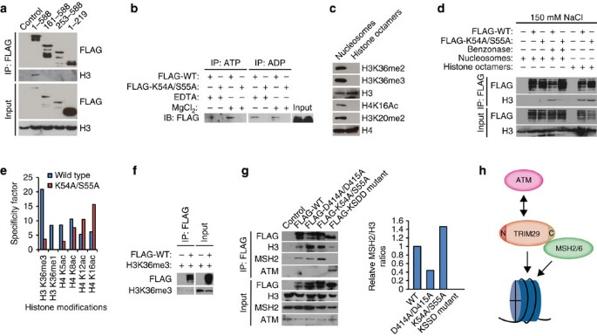Figure 6: TRIM29 directly binds to chromatin. (a) Binding of FLAG-tagged WT TRIM29 and mutants to nucleosomes. Anti-FLAG immunoprecipitates were prepared from nucleosome-enriched nuclear extracts of cells expressing FLAG-tagged WT TRIM29 and truncated mutants. (b) Binding of FLAG-tagged WT TRIM29 and K54A/S55A mutant to ATP and ADP. The assays were performed in the presence of 10 mM MgCl2or 10 mM EDTA. (c) Western blot analysis of mononucleosomes purified from HeLa cells and recombinant human histone octamers with the indicated antibodies to several modified histone proteins. (d) Binding of TRIM29 to nucleosomes purified from HeLa cells and recombinant histone octamers. (e) Binding specificity of FLAG-tagged WT TRIM29 and K54A/S55A mutant to modified histone peptides using Modified Histone Peptide Array. (f) Specific binding of FLAG-tagged WT TRIM29 toX. laevisH3K36me3. (g) Western blot analysis of anti-FLAG immunoprecipitates from nucleosome-enriched nuclear extracts of HeLa S3 cells expressing FLAG-tagged TRIM29 and mutants (K54A/S55A, D414A/D415A and K54A/S55A/D414A/D415A) in which Lys54, Ser55, Asp414 and Asp415 are substituted with Ala. KSDD mutant indicates K54A/S55A/D414A/D415A mutant. (h) Model for the interaction of TRIM29 with MSH2/6, ATM and nucleosomes. Binding of TRIM29 to nucleosomes is dependent on the Walker A motif and on the interaction with MSH2/6. TRIM29 is able to interact with ATM by dissociating from chromatin. Figure 6: TRIM29 directly binds to chromatin. ( a ) Binding of FLAG-tagged WT TRIM29 and mutants to nucleosomes. Anti-FLAG immunoprecipitates were prepared from nucleosome-enriched nuclear extracts of cells expressing FLAG-tagged WT TRIM29 and truncated mutants. ( b ) Binding of FLAG-tagged WT TRIM29 and K54A/S55A mutant to ATP and ADP. The assays were performed in the presence of 10 mM MgCl 2 or 10 mM EDTA. ( c ) Western blot analysis of mononucleosomes purified from HeLa cells and recombinant human histone octamers with the indicated antibodies to several modified histone proteins. ( d ) Binding of TRIM29 to nucleosomes purified from HeLa cells and recombinant histone octamers. ( e ) Binding specificity of FLAG-tagged WT TRIM29 and K54A/S55A mutant to modified histone peptides using Modified Histone Peptide Array. ( f ) Specific binding of FLAG-tagged WT TRIM29 to X. laevis H3K36me3. ( g ) Western blot analysis of anti-FLAG immunoprecipitates from nucleosome-enriched nuclear extracts of HeLa S3 cells expressing FLAG-tagged TRIM29 and mutants (K54A/S55A, D414A/D415A and K54A/S55A/D414A/D415A) in which Lys54, Ser55, Asp414 and Asp415 are substituted with Ala. KSDD mutant indicates K54A/S55A/D414A/D415A mutant. ( h ) Model for the interaction of TRIM29 with MSH2/6, ATM and nucleosomes. Binding of TRIM29 to nucleosomes is dependent on the Walker A motif and on the interaction with MSH2/6. TRIM29 is able to interact with ATM by dissociating from chromatin. Full size image To determine the molecular function of TRIM29, we searched for the functional motif in its N-terminal domain. We found a highly conserved Walker A motif (GXXXXGKS/T) at amino acid residues from 48 to 55 in the N-terminal region ( Supplementary Table 4 ). The Walker A motif is a nucleotide-binding motif that is highly conserved in numerous ATPases [35] . Previous studies revealed that the lysine residue forms a hydrogen bond with oxygen of γ-phosphate of ATP and that the serine/threonine residues interact with Mg ion [36] , [37] . To determine whether TRIM29 has ATP- and ADP-binding abilities, we generated FLAG-TRIM29 WT and a K54A/S55A mutant in which both Lys54 and Ser55 were substituted with Ala. K54A and S55A mutations abrogated the binding of TRIM29 to ATP and ADP ( Fig. 6b ). To determine whether TRIM29 directly binds to histones, we performed an in-vitro binding assay using nucleosomes purified from HeLa cells and recombinant histone octamer. Western blot analysis showed that nucleosomes purified from HeLa cells contained PTMs but that recombinant histone octamer did not ( Fig. 6c ). Intriguingly, a larger amount of TRIM29 bound to nucleosomes treated with benzonase than to non-treated nucleosomes, suggesting that TRIM29 bound to modified histones without assistance of winding DNAs ( Fig. 6d ). K54A/S55A mutation interfered with TRIM29 binding to modified histones, whereas K54A/S55A mutation did not affect TRIM29 interaction with unmodified histones ( Fig. 6d ). To assess the binding specificity of TRIM29 to histone tails, we tested whether TRIM29 binds to specific histone PTMs using modified histone tail peptide arrays. Wild-type TRIM29 exhibited the strongest specificity to H3K36me3 peptide, whereas K54A/S55A mutant did not interact with H3K36me3 peptide. In contrast, K54A/S55A mutant bound to acetylated H4 tail peptides better than did WT TRIM29 ( Fig. 6e ). To investigate the interaction of TRIM29 with recombinant H3K36me3, we performed an in-vitro binding assay using recombinant Xenopus laevis H3K36me3. The in-vitro binding assay showed that TRIM29 directly binds to recombinant H3K36me3 ( Fig. 6f ). These findings indicate that the Walker A motif of TRIM29 regulates the binding of TRIM29 to modified histone tails in the context of nucleosomes. We next tested whether ATP- and MSH2-binding activities of TRIM29 are responsible for chromatin binding. We generated HeLa S3 cells stably expressing FLAG-TRIM29 K54A/S55A, or K54A/S55A/D414A/D415A (KSDD) mutants in which Lys54 and Ser55, or Lys54, Ser55, Asp414 and Asp415 are substituted with Ala, and we prepared nucleosome-enriched extracts from cells expressing the WT or mutants of FLAG-TRIM29. The K54A/S55A and D414A/D415A mutants bound to H3 and MSH2 ( Fig. 6g ). Given that the MSH2-MSH6 dimer directly interacts with chromatin through H3K36me3 (ref. 16 ), residual binding of the D414A/D415A mutant to MSH2 could be due to indirect interaction of TRIM29 with the MSH2-MSH6 dimer through nucleosomes. Consistent with our idea, quadruple mutations diminished the interaction of TRIM29 with MSH2 and H3 ( Fig. 6g ). Interestingly, ATM interacted with the quadruple mutant more strongly than it did with WT TRIM29 and other mutants in the presence of nucleosomes ( Fig. 6g ), indicating that the dissociation of TRIM29 from chromatin is required for its interaction with ATM. Consistent with this observation, TRIM29 interacted with ATM in nuclear extracts prepared by Dignam’s method ( Fig. 1g ). Collectively, our data demonstrate that TRIM29 forms a protein complex with MMR proteins on chromatin and interacts with ATM by its dissociation from chromatin ( Fig. 6h ). Chromatin binding of TRIM29 is required for DDR To investigate the relationship between nuclear localization of TRIM29 and DDR, we treated stably EGFP-TRIM29-expressing HeLa S3 and U2OS cells with 10 Gy IR and analysed the effect of IR treatment on these cells. TRIM29-EGFP in HeLa S3 cells was localized to the nucleus with or without IR treatment ( Fig. 7a ). IR treatment did not cause the translocation of TRIM29-EGFP to the nucleus in U2OS cells ( Fig. 7a ). TRIM29 overexpression in HeLa S3 cells increased the basal level of γH2AX and promoted efficient phosphorylation of H2AX in response to IR treatment, whereas TRIM29 overexpression in U2OS cells suppressed phosphorylation of H2AX in response to IR treatment ( Fig. 7b ). Consistent with these findings, TRIM29-EGFP overexpression rendered U2OS cells to be more radiosensitive ( Fig. 7c ). 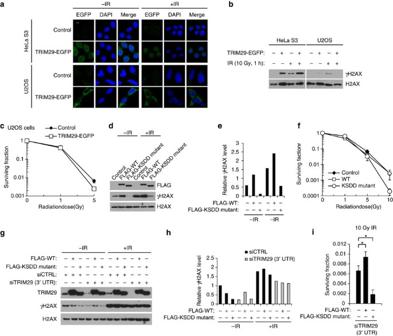Figure 7: Chromatin binding of TRIM29 contributes to efficient activation of DDR. (a) Confocal immunofluorescence images showing the localization of TRIM29-EGFP in HeLa S3 and U2OS cells. Cells were treated with 10 Gy IR and fixed after 1 h. DNA was counterstained with DAPI. Scale bar, 20 μm. (b) Effect of TRIM29 overexpression on histone modifications induced by IR treatment. C-terminal EGFP-tagged TRIM29-expressing HeLa S3 and U2OS cells were treated with 10 Gy IR and collected after 1 h. Proteins were analysed by western blotting using the indicated antibodies. (c) Survival curves of C-terminal EGFP-tagged TRIM29-expressing U2OS cells. Three independent experiments were performed. (d) Effect of point mutations on phosphorylation of H2AX induced by IR treatment. HeLa S3 cells expressing FLAG-tagged WT TRIM29 and K54A/S55A/D414A/D415A mutant were treated with 10 Gy IR and collected after 1 h. Proteins were analysed by western blotting using the indicated antibodies. (e) Effect of the expression of FLAG-tagged WT TRIM29 and K54A/S55A/D414A/D415A mutant on γH2AX induced by IR treatment. The intensities of γH2AX were normalized with the values of H2AX. (f) Survival curves of FLAG-tagged WT TRIM29 and K54A/S55A/D414A/D415A mutant-expressing HeLa S3 cells. Three independent experiments were performed. (g) Western blotting of FLAG-tagged WT TRIM29 and KSDD mutant-expressing HeLa S3 cells transfected with the indicated siRNAs. Cells were transfected with siCTRL or siTRIM29 targeting the 3′-UTR ofTRIM29mRNA. After 72 h, cells were treated with 10 Gy IR and collected after 1 h. Proteins were analysed by western blotting using the indicated antibodies. (h) Effect of TRIM29 knockdown on γH2AX induced by IR treatment. The intensities of γH2AX were normalized with the values of H2AX. (i) Effect of TRIM29 knockdown on cell viability in response to IR treatment. FLAG-tagged WT TRIM29 and KSDD mutant-expressing HeLa S3 cells were transfected with siCTRL or siTRIM29 targeting the 3′-UTR ofTRIM29mRNA. After 72 h, cell viability in response to IR treatment was analysed by a colony-formation assay.P-values were determined by Student’st-test (*P<0.05). Three independent experiments were performed. Error bars show s.d. Figure 7: Chromatin binding of TRIM29 contributes to efficient activation of DDR. ( a ) Confocal immunofluorescence images showing the localization of TRIM29-EGFP in HeLa S3 and U2OS cells. Cells were treated with 10 Gy IR and fixed after 1 h. DNA was counterstained with DAPI. Scale bar, 20 μm. ( b ) Effect of TRIM29 overexpression on histone modifications induced by IR treatment. C-terminal EGFP-tagged TRIM29-expressing HeLa S3 and U2OS cells were treated with 10 Gy IR and collected after 1 h. Proteins were analysed by western blotting using the indicated antibodies. ( c ) Survival curves of C-terminal EGFP-tagged TRIM29-expressing U2OS cells. Three independent experiments were performed. ( d ) Effect of point mutations on phosphorylation of H2AX induced by IR treatment. HeLa S3 cells expressing FLAG-tagged WT TRIM29 and K54A/S55A/D414A/D415A mutant were treated with 10 Gy IR and collected after 1 h. Proteins were analysed by western blotting using the indicated antibodies. ( e ) Effect of the expression of FLAG-tagged WT TRIM29 and K54A/S55A/D414A/D415A mutant on γH2AX induced by IR treatment. The intensities of γH2AX were normalized with the values of H2AX. ( f ) Survival curves of FLAG-tagged WT TRIM29 and K54A/S55A/D414A/D415A mutant-expressing HeLa S3 cells. Three independent experiments were performed. ( g ) Western blotting of FLAG-tagged WT TRIM29 and KSDD mutant-expressing HeLa S3 cells transfected with the indicated siRNAs. Cells were transfected with siCTRL or siTRIM29 targeting the 3′-UTR of TRIM29 mRNA. After 72 h, cells were treated with 10 Gy IR and collected after 1 h. Proteins were analysed by western blotting using the indicated antibodies. ( h ) Effect of TRIM29 knockdown on γH2AX induced by IR treatment. The intensities of γH2AX were normalized with the values of H2AX. ( i ) Effect of TRIM29 knockdown on cell viability in response to IR treatment. FLAG-tagged WT TRIM29 and KSDD mutant-expressing HeLa S3 cells were transfected with siCTRL or siTRIM29 targeting the 3′-UTR of TRIM29 mRNA. After 72 h, cell viability in response to IR treatment was analysed by a colony-formation assay. P -values were determined by Student’s t -test (* P <0.05). Three independent experiments were performed. Error bars show s.d. Full size image The KSDD mutant interacted with ATM but not with nucleosomes ( Fig. 6h ). To determine whether the interaction of TRIM29 with chromatin is needed to activate DDR, we investigated the effect of overexpression of WT TRIM29 and KSDD mutant on the induction of γH2AX and the radioresistance of cells. Overexpression of TRIM29 increased the basal level of γH2AX and the level of IR-induced γH2AX ( Fig. 7d,e ). Even in the presence of endogenous TRIM29, the KSDD mutant had a dominant-negative effect on the basal level of γH2AX and the level of IR-induced γH2AX ( Fig. 7d,e ). Overexpression of WT TRIM29 had little effect on the radioresistance ( Fig. 7f ). Notably, overexpression of the KSDD mutant reduced the radioresistance of cells to an extent similar to that by TRIM29 knockdown ( Fig. 7f ). As the KSDD mutant is able to interact with ATM but not with nucleosomes ( Fig. 6h ), the KSDD mutant may elicit a dominant-negative effect on DDR by inhibiting the binding of ATM to chromatin. To reduce the effect of endogenous TRIM29, WT FLAG-TRIM29 or KSDD mutant-expressing HeLa S3 cells were transfected with siRNA targeting the 3′-untranslated region (UTR) of TRIM29 messenger RNA. Even in the presence of endogenous TRIM29, the KSDD mutant had a dominant-negative effect on the basal level of γH2AX ( Fig. 7g,h ). In the absence of endogenous TRIM29, the basal level of γH2AX was increased by WT TRIM29 but not by the KSDD mutant ( Fig. 7g,h ), indicating that TRIM29 is required for the basal level of γH2AX induced by spontaneous DNA damage. Furthermore, overexpression of WT TRIM29 increased the radioresistance of cells, whereas the KSDD mutant failed to contribute to the radioresistance of cells ( Fig. 7i ). These findings suggest that chromatin binding of TRIM29 enhances DDR by mediating the interaction of DNA repair proteins with chromatin. Functional relationship between TRIM29 and MSH2 We investigated the potential role of MSH2 in binding of TRIM29 to chromatin and DNA repair proteins. To examine whether MSH2 regulates the chromatin association of TRIM29, we depleted HeLa S3 cells of MSH2 by siRNA transfection and then fractionated the lysates of the cells into cytoplasmic, nucleoplasmic and chromatin fractions as shown in Fig. 1a [28] . MSH2 depletion did not alter the chromatin association of endogenous TRIM29 and FLAG-TRIM29 ( Fig. 8a,b ). We next examined whether MSH2 is a critical linker between TRIM29 and ATM. We depleted stably FLAG-TRIM29-expressing HeLa S3 cells of MSH2 by siRNA transfection and then we prepared nuclear extracts from siRNA-treated cells and analysed the binding of TRIM29 to ATM. As shown in silver staining of the TRIM29 complex, knockdown of MSH2 had no effect on the overall composition of the complex ( Fig. 8c ) and did not significantly decrease the interaction of TRIM29 with ATM; however, the interaction of TRIM29 with MLH1 was abrogated by MSH2 depletion ( Fig. 8d ). These findings indicate that TRIM29 binds to MMR proteins through MSH2, but that TRIM29 binds to ATM probably through other components of the TRIM29 complex. 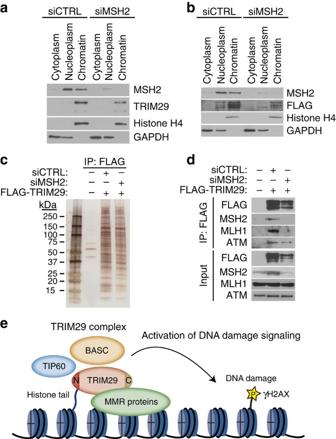Figure 8: MSH2 is a critical linker between TRIM29 and DNA MMR proteins. (a) Effect of MSH2 knockdown on chromatin association of endogenous TRIM29 in HeLa S3 cells. HeLa S3 cells were transfected with siControl or siMSH2 and incubated for 48 h. Total proteins (10 μg) from cytoplasm, nucleoplasm and chromatin fractions were subjected to SDS–PAGE followed by western blotting. (b) Effect of MSH2 knockdown on chromatin association of FLAG-tagged TRIM29 in HeLa S3 cells. HeLa S3 cells stably expressing FLAG-tagged TRIM29 were transfected with siControl or siMSH2 and incubated for 48 h. Total proteins (10 μg) from the cytoplasm, nucleoplasm and chromatin fractions were subjected to SDS–PAGE followed by western blotting. (c) Silver staining of anti-FLAG immunoprecipitates from nuclear extracts of MSH2-depleted cells expressing FLAG-tagged TRIM29 on 4%–20% gradient SDS–PAGE gel. (d) Interaction of FLAG-TRIM29 with ATM. HeLa S3 cells stably expressing FLAG-tagged TRIM29 were transfected with siControl or siMSH2. After 48 h, nuclear extracts were prepared from each cell line. Anti-FLAG immunoprecipitates were prepared from nuclear extracts and analysed by western blotting. (e) Model for TRIM29 function in activation of DNA damage signalling. TRIM29 binds to modified histone tails and functions as a molecular scaffold with DNA MMR proteins. These interactions are responsible for efficient activation of DDR. The assembly of TRIM29 and DNA repair proteins into chromatin is dependent on pre-existing H3K36me2, H4K16Ac and H4K20me2. Figure 8: MSH2 is a critical linker between TRIM29 and DNA MMR proteins. ( a ) Effect of MSH2 knockdown on chromatin association of endogenous TRIM29 in HeLa S3 cells. HeLa S3 cells were transfected with siControl or siMSH2 and incubated for 48 h. Total proteins (10 μg) from cytoplasm, nucleoplasm and chromatin fractions were subjected to SDS–PAGE followed by western blotting. ( b ) Effect of MSH2 knockdown on chromatin association of FLAG-tagged TRIM29 in HeLa S3 cells. HeLa S3 cells stably expressing FLAG-tagged TRIM29 were transfected with siControl or siMSH2 and incubated for 48 h. Total proteins (10 μg) from the cytoplasm, nucleoplasm and chromatin fractions were subjected to SDS–PAGE followed by western blotting. ( c ) Silver staining of anti-FLAG immunoprecipitates from nuclear extracts of MSH2-depleted cells expressing FLAG-tagged TRIM29 on 4%–20% gradient SDS–PAGE gel. ( d ) Interaction of FLAG-TRIM29 with ATM. HeLa S3 cells stably expressing FLAG-tagged TRIM29 were transfected with siControl or siMSH2. After 48 h, nuclear extracts were prepared from each cell line. Anti-FLAG immunoprecipitates were prepared from nuclear extracts and analysed by western blotting. ( e ) Model for TRIM29 function in activation of DNA damage signalling. TRIM29 binds to modified histone tails and functions as a molecular scaffold with DNA MMR proteins. These interactions are responsible for efficient activation of DDR. The assembly of TRIM29 and DNA repair proteins into chromatin is dependent on pre-existing H3K36me2, H4K16Ac and H4K20me2. Full size image Many of the chromatin-associated proteins have an ATP-dependent function [38] . To examine whether interaction of the TRIM29–MSH2 complex with chromatin is dependent on ATP in cells, we examined the effects of ATP and ATPγS on binding of the TRIM29–MSH2 complex and nucleosomes. ATP did not alter the binding of the TRIM29–MSH2 complex to histone H3 ( Supplementary Fig. 5a ), whereas ATPγS abrogated the interaction of the TRIM29–MSH2 complex with H3 ( Supplementary Fig. 5b ). These findings suggest that interaction of the TRIM29–MSH2 complex with chromatin is dependent on ATP hydrolysis. Taken together, the findings indicate that chromatin binding of TRIM29 has a major role in the activation of DNA damage signalling. We propose a model in which TRIM29 forms a molecular scaffold with MMR proteins on chromatin and mediates the interaction between DNA repair proteins and chromatin ( Fig. 8e ). In this study, we showed that TRIM29 is a histone-binding protein involved in the incorporation of DNA repair proteins into chromatin ( Fig. 8e ). TRIM29 is one of the components of the DNA repair complex composed of BASC, cohesion, DNA-PKcs and TIP60 complex. These proteins function in distinct cellular events including DNA replication, DNA repair and transcription, but they share the function in the DSB repair system. Among these DNA repair proteins, TRIM29 directly binds to MSH2. It has been reported that MMR proteins including MSH2 function as molecular scaffolds to regulate ATM activity and regulate the recruitment of MRE11 to DSB sites [39] , [40] . Consistent with these findings, we revealed that TRIM29 forms a scaffold structure with DNA MMR proteins on chromatin to regulate DNA damage signalling. Intriguingly, there are chromatin-bound and unbound forms of TRIM29 ( Figs 1g , 6h ). We also revealed that the chromatin-unbound form of TRIM29 can tightly interact with ATM and acts as a dominant-negative form in cell survival ( Figs 6h , 7f ). There is a possibility that chromatin binding of TRIM29 is regulated by ATM in response to DNA damage. In agreement with this speculation, a recent study showed that TRIM29 is phosphorylated by ATM in response to IR [22] . The functional relationship between chromatin binding of TRIM29 and the function of ATM remains to be investigated. Our biochemical studies demonstrated that TRIM29 directly binds to modified histone tails in the context of nucleosomes. Histone peptide array analysis showed that TRIM29 preferentially binds to H3K36me3 and modified H4 tails. We further showed that chromatin binding of TRIM29 is responsible for the activation of DDR. These findings provide evidence that TRIM29 regulates DDR by interacting with modified histone tails. Chromatin-associated proteins recognize histone PTMs through the PTM-reading domain [41] . Thus, TRIM29 may have a functional domain responsible for binding to histones. Histone PTMs play a prominent role in the accumulation of DNA repair proteins at DNA damage sites [11] . We showed that pre-existing H3K36me2, H4K16Ac and H4K20me2 are required for assembly of the TRIM29 complex into H2AX-containing histones. The importance of pre-existing H3K36me2 on H2AX nucleosomes is consistent with the results of a previous study showing that H3K36me2 enhances recruitment of the MRN complex to DSB sites [14] . TIP60-dependent H4K16Ac inhibits the binding of 53BP1 to chromatin and promotes the accumulation of BRCA1 at DSB sites [13] , indicating that incorporation of TIP60 into the TRIM29-containing complex may contribute to the accumulation of BASC at nucleosomes containing H2AX. In contrast to the pre-existing H3K36me2, H4K16Ac and H4K20me2 on H2AX-containing nucleosomes, induction of H3K36me3 is also accompanied by reduction of H4K16Ac and H4K20me2 on nucleosomes containing H2AX. SETD2-dependent H3K36me3 has recently been shown to facilitate the recruitment of RAD51 to DSB sites [15] , [17] . We have already identified SETD2 as a TRIM29-binding protein by MudPIT mass spectrometry ( Supplementary Table 1 ), suggesting that SETD2-dependent H3K36me3 regulates the incorporation of TRIM29 and DNA repair proteins into damaged chromatin. TRIM29 does not accumulate at γH2AX foci in response to DSBs. Several DNA repair proteins do not accumulate at IR-induced DSBs. DNA-PKcs, Ku70, SMC1, SMC3 and hnRNPUL1/2 have been reported to be undetectable in IR-induced foci, because only a small amount of proteins is presumably recruited to IR-induced foci [42] , [43] , [44] . It is possible that we were unable to detect the accumulation of TRIM29 at DSB sites for the same reason. Interestingly, TRIM29 dissociates from γH2AX in response to DSBs. It has recently been reported that THRAP3, hnRNPUL proteins 1/2 and SAFB1 are rapidly recruited to DNA damage sites, and that they are then excluded from damaged chromatin and efficiently promote DNA damage signalling [44] , [45] , [46] . Transient recruitment followed by exclusion from DSB sites is an emerging mechanism involved in the maintenance of genome stability. Given the dissociation of TRIM29 from γH2AX after DNA damage, TRIM29 may function in the same mechanism as these proteins. As TRIM29 has histone-binding activity, the localization of TRIM29 on chromatin should be a characteristic common to all cell lines. However, subcellular localization of TRIM29 depended on the cell type. This discrepancy in the subcellular localization of TRIM29 indicates that there is a certain factor that regulates the chromatin localization of TRIM29. A recent study showed that phosphorylation of TRIM29 by MK2 contributes to the radioresistance of cells [22] . The phosphorylation of TRIM29 by MK2 may be associated with nuclear localization of TRIM29. It is important to clarify the mechanism underlying the subcellular localization of TRIM29 in the future. Our study demonstrated that TRIM29 assembles DNA repair proteins into chromatin. Functional interactions among TRIM29, DNA repair proteins and chromatin may be required for activating the DNA repair pathway. The dynamics of DNA repair proteins through TRIM29–histone PTM interaction might control a cellular response to genotoxic stress. It is important to clarify how TRIM29 recognizes histone PTMs, how TRIM29 regulates the function of DNA repair proteins on chromatin and how these steps promote DNA damage signalling. Plasmids Full-length human TRIM29 (NM_012101.3), MSH2 (NM_000251.2), DMAP1 (NM_019100.4), ING3 (NM_019071.2) and H2AX (NM_002105.2) were amplified using total RNA from HeLa cells. Human TIP60 complementary DNA was kindly provided by Dr Ikura (Kyoto University). Cell culture HEK293T, HeLa, HeLa S3 and SiHa cell lines were cultured in DMEM (Sigma-Aldrich Corp., St Louis, MO) supplemented with 10% fetal bovine serum (FBS). U2OS cells were cultured McCoy’s medium (Sigma) supplemented with 10% FBS (Invitrogen, Carlsbad, CA). All cell lines were cultured under an atmosphere of 5% CO 2 at 37 °C. For large-scale culture, parental HeLa S3 cells and their derivatives were cultured in spinner culture in Joklik’s medium (Sigma) with 5% calf serum (Invitrogen) [30] . Recombinant protein and reagent Mouse anti-FLAG M2 was from Sigma (1:2,000 dilutions). Mouse anti-TRIM29 (1:100 dilutions, sc-166718) were from Santa Cruz Biotechnology (Santa Cruz, CA). Rabbit anti-H4K20me2 (1:1,000 dilutions, 9,759), rabbit anti-histone H3 (1:1,000 dilutions, 4,499), mouse anti-MLH1 (1:1,000 dilutions, 3,515), rabbit anti-MSH2 (1:1,000 dilutions, 2,017), rabbit anti-MSH6 (1:1,000 dilutions, 3,996), rabbit anti-ATM (1:1,000 dilutions, 2,873), rabbit anti-H3K27me3 (1:1,000 dilutions, 9,733), rabbit anti-GST (1:1,000 dilutions, 2,622), rabbit anti-histone H2A (1:1,000 dilutions, 2,578), rabbit anti-H2AK5Ac (1:1,000 dilutions, 2,576), rabbit anti-H2AK119Ub (1:1,000 dilutions, 8,240), rabbit anti-γH2AX (1:1,000 dilutions, 9,718), rabbit anti-RUVBL1 (1:1,000 dilutions, 12,300), rabbit anti-H4K5Ac (1:1,000 dilutions, 9,672), rabbit anti-H4K8Ac (1:1,000 dilutions, 2,594), rabbit anti-H4K12Ac (1:1,000 dilutions, 2,591) and rabbit anti-H4K16Ac (1:1,000 dilutions, 8,804) were from Cell Signaling Technology (Beverly, MA). Rabbit anti-TIP60 (1:1,000 dilutions, 07-038) and rabbit anti-H3K9me3 (1:1,000 dilutions, 07-523) were from Millipore (Temecula, CA). Mouse anti-BRCA1 (1:1,000 dilutions, ab16780), rabbit anti-DNA-PKcs (1:1,000 dilutions, ab32566), rabbit anti-histone H2AX (1:1,000 dilutions, ab11175), rabbit anti-histone H4 (1:1,000 dilutions, ab10158), rabbit anti-H3K36me3 (1:1,000 dilutions, ab9050), rabbit anti-BAF53 (1:1,000 dilutions, ab3883) and rabbit anti-ING3 (1:1,000 dilutions, ab84645) were from Abcam (Cambridge, UK). Rabbit anti-SMC1 (1:1,000 dilutions, A300-055A) and rabbit anti-SMC3 (1:1,000 dilutions, A300-060A) were from Bethyl Laboratories (Montgomery, TX). Mouse anti-GAPDH (AM4300) was from Ambion (Austin, TX). Alexa Fluor 488-labelled anti-mouse IgG (1:1,000 dilutions) and goat Alexa Fluor 555-labelled anti-rabbit IgG antibody (1:1,000 dilutions) were from Invitrogen. Recombinant human MSH2 protein (P01) was purchased from Abnova (Taipei, Taiwan). Recombinant human histone octamer (16-0001) and HeLa-purified mononucleosomes (16-0002) were purchased from EpiCypher (The Woodlands, TX). Recombinant X. laevis histone H3K36me3 (MLA) was purchased from Active Motif (Carlsbad, CA). MNNG was from Tokyo Kasei Kogyo (Tokyo, Japan). Subcellular fractionation HeLa S3, HeLa and SiHa cells were grown in large-scale suspension cultures or cultured in a 100-mm plastic dish (Corning 430167; Corning Co., NY, USA). The cells were lysed with cytoplasmic lysis buffer (10 mM Hepes buffer (pH 7.9) containing 0.34 M sucrose, 3 mM CaCl 2 , 2 mM MgAc, 0.1 mM EDTA, 1 mM dithiothreitol (DTT), 0.5% (v/v) NP-40 and Protease Inhibitor Cocktail (Complete, EDTA-free; Roche)). Intact nuclei were pelleted by centrifugation at 2,600 g for 15 min and washed with cytoplasmic lysis buffer without NP-40. Nuclei were then lysed with nuclear lysis buffer (20 mM Hepes buffer (pH 7.9) containing 3 mM EDTA, 10% (v/v) glycerol, 150 mM KAc, 1.5 mM MgCl 2 , 1 mM DTT, 0.1% (v/v) NP-40 and Protease Inhibitor Cocktail). The nucleoplasmic fraction was cleared by centrifugation at 27,000 g for 30 min. The chromatin pellet was suspended in nuclease incubation buffer (150 mM Hepes buffer (pH 7.9) containing 1.5 mM MgCl 2 , 150 mM KAc, 10% (v/v) glycerol and Protease Inhibitor Cocktail). Digestion of DNA and RNA in the suspension with 0.15 unit per μl benzonase (Sigma) was performed at 4 °C for 1 h. The chromatin fraction was cleared by centrifugation at 100,000 g for 30 min. Generation of stable cell lines cDNAs encoding full-length WT and various mutant versions of TRIM29, MSH2, TIP60, DMAP1 and ING3 were introduced by retroviral transduction into a HeLa S3 cell line stably expressing the mouse ectopic retrovirus receptor (mCAT-1) [47] . Retroviruses were produced with Plat-E packaging cells [48] . Nuclear extracts of HeLa S3 cells expressing FLAG-tagged proteins expressing HeLa S3 cells were prepared according to Dignam’s method [49] . Immunoprecipitation and affinity purification Protein complexes were purified from nuclear extracts of cells stably expressing FLAG-tagged proteins as described below. Nuclear extracts were incubated with anti-FLAG agarose beads (50 μl per 1 mg of nuclear extract) for 2 h at 4 °C. The beads were then washed five times with 50 mM Hepes buffer (pH 7.9) containing 0.3 M NaCl, 0.1% (v/v) Triton X-100 and 10 mM MgCl 2 . The binding proteins were then eluted by 3 × FLAG peptides (250 ng μl −1 ) in 50 mM Hepes buffer (pH 7.9) containing 100 mM NaCl, 0.1 mM EDTA (pH 8.0), 0.1% (v/v) Triton X-100 and 10% (v/v) glycerol. Uncropped immunoblots are available in Supplementary Figs 6–20 . Mass spectrometry Proteins were identified using MudPIT. NSAFs were used to estimate relative protein abundance [30] . Recombinant protein production FLAG-tagged TRIM29 and HA-tagged full-length and deletion mutants of MSH2 in the pCold-ProS2 vector (Takara, Shiga, Japan) were expressed in BL21 (DE3) cells and purified using ProBond Ni-Cheleting Resin (Life Technologies, Gaithersburg, MD) as described in the instruction manual. His-ProS2-FLAG-tagged TRIM29 was digested by HRV 3C Protease (Takara) in 50 mM Hepes buffer (pH 7.9) containing 150 mM NaCl. FLAG-tagged TRIM29 was purified by removing the His-ProS2 tag using ProBond Ni-Cheleting Resin and was stored in 50 mM Hepes buffer (pH 7.9) containing 150 mM NaCl and 10% (v/v) glycerol. For production of FLAG-tagged WT and mutants of TRIM29 in Sf9 cells, FLAG-tagged WT TRIM29 and mutant were subcloned into the pFastBac HTa vector. Sf9 insect cells were cultured at 28 °C in Sf-900 II SFM (Invitrogen) supplemented with 10% FBS. Sf9 cells infected with a recombinant baculovirus were lysed in 50 mM Hepes buffer (pH 7.9) containing 150 mM NaCl, 10% glycerol and 1% Triton X-100. In-vitro binding assay WT FLAG-tagged TRIM29 and the mutant were bound to M2-agarose (Sigma) in binding buffer (50 mM Hepes buffer (pH 7.9), 150 mM NaCl, 0.1% (v/v) Triton X-100 and 10% (v/v) glycerol). GST-MSH2, His-ProS2-HA-taggged deletion mutants of MSH2, mononucleosomes purified from HeLa cells and histone octamer were then added to the bead and incubated at 4 °C for 1 h. M2-agaroses were then washed five times with a binding buffer. The binding proteins were then eluted by 3 × FLAG peptides (250 ng μl −1 ) in a binding buffer. ATP- and ADP-binding assay FLAG-tagged WT TRIM29 and mutant were incubated with ATP- or ADP-agarose (Sigma) at 30 °C for 30 min in binding buffers (50 mM Hepes buffer (pH 7.9), 150 mM NaCl, 0.1% (v/v) Triton X-100 and 10% (v/v) glycerol) containing 10 mM MgCl 2 or 10 mM EDTA. The bound proteins were washed by each binding buffer and then eluted by 2 mM ATP in binding buffer. Nucleosome pull-down assay We prepared nuclei pellets from HeLa S3 cells expressing FLAG-tagged WT TRIM29 and mutants according to Dignam’s method [49] . The nuclei pellets were suspended in MNase reaction buffer (micrococcal nuclease (100 U ml −1 ; Takara), complete protease inhibitor cocktail, EDTA-free (Roche), 50 mM Hepes buffer (pH 7.9), 5 mM MgCl 2 , 5 mM CaCl 2 and 25% (v/v) glycerol) and incubated for 10 min at room temperature. The nucleosome-enriched nuclear extract was cleared by centrifugation for 30 min at 100,000 g . Fifty microlitres of M2-agarose (Sigma) were added to 10 mg nucleosome-enriched extracts and incubated at 4 °C for 1 h. M2-agaroses were then washed five times with a binding buffer (50 mM Hepes buffer (pH 7.9), 5 mM MgCl 2 , 5 mM CaCl 2 , 0.1% (v/v) Triton X-100 and 10% (v/v) glycerol) containing 0–500 mM NaCl. The binding proteins were then eluted by 3 × FLAG peptides (250 ng μl −1 ) in a binding buffer (20 mM Hepes buffer (pH 7.9), 100 mM NaCl, 0.1 mM EDTA (8.0), 0.05% (v/v) Triton X-100 and 10% (v/v) glycerol). Histone peptide array A modified histone peptide array (Active Motif) was blocked in TBST buffer (20 mM Tris-HCl buffer (pH 8.0), 150 mM NaCl and 0.05% (v/v) Tween-20) containing 10% (w/v) non-fat dried milk at 4 °C overnight. The array was then washed three times for 5 min each time with TBST. Proteins were incubated with the arrays at 4 °C overnight in an interaction buffer (20 mM Hepes buffer (pH 7.9), 300 mM NaCl, 1.5 mM MgCl 2 , 0.1% (v/v) Triton X-100). After washing three times for 5 min each time with TBST, the array was incubated with mouse anti-TRIM29 at 4 °C overnight. The array was then washed three times for 5 min each time with TBST and incubated with a secondary antibody in TBST containing 3% (w/v) non-fat dried milk for 1 h at room temperature. The array was submerged in enhanced chemiluminescence developing solution. Images were captured on film and the data were analysed using array analyser software (Active Motif). siRNA transfections HeLa S3 cells in six-well tissue culture plates ( ∼ 1 × 10 5 cells per well) or 10-cm dishes ( ∼ 2 × 10 6 cells per dish) were transfected with 25 nM siRNA ON-TARGETplus human TRIM29 siRNA SMART pool (Dharmacon, Pittsburgh, PA) or 25 nM siGENOME NON-TARGETING siRNA Pool #2 (Dharmacon) using Lipofectamine RNAi MAX (Invitrogen). After 48 h of culture, cells were subjected to each analysis. Parental HeLa S3 cells and their derivatives in six-well tissue culture plates ( ∼ 1 × 10 5 cells per well) were transfected with 1 μM Accell Non-targeting Pool (Dharmacon) or Accell Human TRIM29 (23650) siRNA Individual (Dharmacon) targeting 3′-UTR of TRIM29 mRNA. After 72 h of culture, cells were subjected to each analysis. Immunostaining Cells were cultured on a cover glass in DMEM supplemented with 10% FBS under an atmosphere of 5% CO 2 at 37 °C. The cells were treated with nuclear extraction buffer (20 mM Hepes buffer (pH 7.9) containing 20 mM NaCl, 5 mM MgCl 2 , 1 mM DTT, 0.5% (v/v) NP-40, Phosphatase Inhibitor Cocktail (Sigma) and Protease Inhibitor Cocktail) for 20 min at 4 °C. Next, the cells were fixed with 4% paraformaldehyde in PBS for 15 min at room temperature, washed with PBS three times and incubated with blocking buffer (5% normal goat serum and 0.1% Triton X-100 in PBS) for 1 h. After blocking, the cells were incubated with primary antibodies in blocking buffer overnight at 4 °C and incubated with goat Alexa Fluor 488-labelled anti-mouse IgG (1:1,000 dilutions) or goat Alexa Fluor 555-labelled anti-rabbit IgG antibody (1:1,000 dilutions) for 1 h at room temperature. DNA was counterstained with 0.4 μg ml −1 DAPI in PBS for 30 min at room temperature. Confocal images were taken using an upright microscope (FV1000, Olympus, Tokyo, Japan). γH2AX foci were quantified by CellProfiler software ( http://www.cellprofiler.org ). Clonogenic survival assay Cells were diluted to the desired concentration and attached to six-well plates. The cells were irradiated with increasing doses of IR or exposed to 10 μM MNNG for 2 h. After 10–14 days, cells were fixed with 4% paraformaldehyde in PBS for 15 min at room temperature and stained with 1% crystal violet in ethanol. Colonies with more than 50 cells were counted. Plating efficiency was calculated as the ratio of the number of colonies to the number of cells cultured. Surviving fraction was normalized to plating efficiency. Three independent experiments were performed. Irradiation Irradiation (125 kVp, 15 mA, 0.5 mm aluminium and 0.1 mm copper filters) was performed using X-ray irradiation equipment MBR-1520R-3 (Hitachi, Tokyo, Japan). How to cite this article : Masuda, Y. et al. TRIM29 regulates the assembly of DNA repair proteins into damaged chromatin. Nat. Commun. 6:7299 doi: 10.1038/ncomms8299 (2015).